Electrical power generation by mechanically modulating electrical double layers Since Michael Faraday and Joseph Henry made their great discovery of electromagnetic induction, there have been continuous developments in electrical power generation. Most people today get electricity from thermal, hydroelectric, or nuclear power generation systems, which use this electromagnetic induction phenomenon. Here we propose a new method for electrical power generation, without using electromagnetic induction, by mechanically modulating the electrical double layers at the interfacial areas of a water bridge between two conducting plates. We find that when the height of the water bridge is mechanically modulated, the electrical double layer capacitors formed on the two interfacial areas are continuously charged and discharged at different phases from each other, thus generating an AC electric current across the plates. We use a resistor-capacitor circuit model to explain the results of this experiment. This observation could be useful for constructing a micro-fluidic power generation system in the near future. Most objects in contact with water or an aqueous solution acquire some electronic charges on their surfaces. These charges on the surface attract counter ions from the liquid, which electrically screen the surface charges. However, owing to thermal energy effects, these counter ions are not firmly anchored to the surface. Instead, they are distributed near the surface, with an exponential decrease in the electrical potential with increasing distance from the surface. This complex system is called an electrical double layer (EDL) [1] , [2] , [3] , [4] , [5] . As its geometry and structure are similar to an electric capacitor, it is also called an electrical double layer capacitor (EDLC) [6] , [7] , [8] . Numerous studies of the EDL have explained many electrokinetic phenomena [9] , [10] , such as, electro-osmosis, electrophoresis and streaming current. There is one prior approach, which uses a streaming current, to generate electrical energy in micro-fluidic channels [11] , [12] . A drawback of this technique is that a continuous pressure gradient must be maintained across the channel in order to generate an electrical current. Recently, a new approach has been suggested for generating electrical energy in micro-fluidic systems [13] using reverse electrowetting [14] . In this technique, the electrons, supplied by an external DC bias-voltage source, act as charge carriers inside a liquid metal (Galinstan, Mercury). External vibration makes the complex system of a liquid metal droplet and two electrodes, where one of them has a dielectric coating on the surface, behave as one variable capacitor where external periodic work is converted to electrical energy. Here, we propose a new method of AC electrical power generation by using plain water, without the need for any external bias-voltage source. In this technique, the ions in the water act as charge carriers inside a water droplet. When a water bridge is formed between two conducting plates, this system behaves as two serially connected electric double layer capacitors. We find that when the height of the water bridge is mechanically modulated, the two capacitors formed on the two interfacial areas are continuously charged and discharged at different phases from each other, thus generating an AC electric current across the plates. A simple resistor-capacitor circuit model and a dimensionless relaxation time are used to explain the results of the experiment. The maximum size of each water bridge is limited by the capillary length of water. This difficulty can be overcome by forming numerous small and equally sized water bridges in parallel between the two plates in order to increase the power generation. In this experiment, roughly 1 ml of water can generate about 1.5 μW of the power and the maximum power density is 0.3 μW cm −2 . 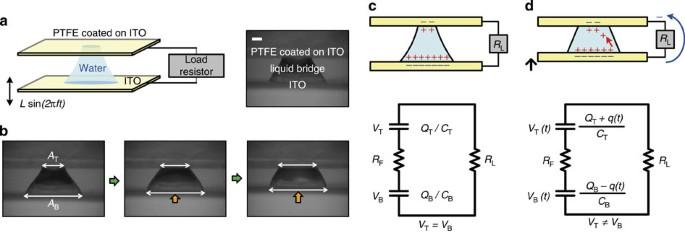Figure 1: Schematic diagram of the experiment and resistor-capacitor circuit model. (a) Experimental setup and (b) video images of water bridge over time. Scale bar, 1 mm. Charge distributions on EDLCs and corresponding equivalent electrical circuits (c) when the water bridge height is fixed in time (equilibrium state) and (d) at the very moment when the two plates are approaching each other (non-equilibrium state). Within a couple of periods after the vibration starts, the system reaches a steady state. Modulating electrical double layers Figure 1a shows a schematic diagram of the experiment. A water bridge is positioned between two parallel conducting plates, where the distance between the plates is mechanically modulated by vertically vibrating the bottom plate in accordance with the form of L sin( 2 π ft ). When the voltage drop across the load resistance R L is measured, an electrical current is observed. The difference in the two contact areas between the water and two conducting plates has a key role in the generation of this electrical current. Therefore, to conduct a controlled and systematic study of this unusual observation, the wetting properties of two conducting plates are made quite different from each other. In this experiment, the top plate is hydrophobic, whereas the bottom plate is hydrophilic. The contact area A B between the water and bottom plate does not change appreciably during the oscillation period due to the small contact angle and pinning effects [15] . In contrast to this, the contact area A T between the water and top plate changes appreciably during each oscillation period ( Fig. 1b ) due to the hydrophobic nature of this plate. Here, we assume that the capacitances ( C T , C B ) of both top and bottom EDLCs increase linearly with the contact areas ( A T , A B ) where Figure 1: Schematic diagram of the experiment and resistor-capacitor circuit model. ( a ) Experimental setup and ( b ) video images of water bridge over time. Scale bar, 1 mm. Charge distributions on EDLCs and corresponding equivalent electrical circuits ( c ) when the water bridge height is fixed in time (equilibrium state) and ( d ) at the very moment when the two plates are approaching each other (non-equilibrium state). Within a couple of periods after the vibration starts, the system reaches a steady state. Full size image Here, d is the thickness of the PTFE coating on the ITO surface of the top plate, λ D is the width of the top EDL, ε p is the dielectric constant of the PTFE, and ε d is the dielectric constant of a water droplet. As d / ε p >> λ D / ε d in this experiment, the first approximation in equation (1) can be justified [16] , [17] . Resistor-capacitor circuit model Under these assumptions, it is possible to express the electrical current flowing in Fig. 1a using a simple equivalent electrical circuit. Figure 1c is the electrical circuit for the case where a long time has passed as the formation of the water bridge and the distance between the plates is constant over time. Here, V T ( Q T ) and V B ( Q B ) are the voltages (charges stored) on C T and C B , respectively, where V T =Q T / C T and V B = Q B / C B . R F is the electrical resistance across the water bridge. As the system is fully relaxed, V T = V B and no current flows. Figure 1d shows the electrical circuit at the very moment when the two plates are approaching each other immediately after the vibration commences at t= 0. In this case, as the contact area at the bottom (top) plate is fixed (increasing), C B is fixed and C T is increasing. Therefore, it is possible to express the electric circuit, shown in Fig. 1d , by using the following differential equation. Here, q ( t ) is the increment (decrement) of charge in the top (bottom) EDLC at time t . This movement of charge between the two capacitors occurs until V T = V B because of the relaxation process. As C T ( t ) increases in time, as depicted in Fig. 1d , the voltage V T ( t ) on the top ELDC decreases, which generates a voltage difference, ΔV≡V B ( t )− V T ( t ), across the plates. In this non-equilibrium state, electrical current flows. Therefore, there is electrical charging ( q ( t )>0) in the top EDLC, with simultaneous electrical discharging in the bottom EDLC. If the distance between the two plates is oscillating at frequency f , the EDLCs formed on the two interfacial areas continuously charge and discharge at different phases relative to each other, which generates an AC electrical current dq/ d t . The voltage drop on R L is V L ( t ) =ΔV ( t ) R L /( R F +R L ). The six graphs in Fig. 2 depict the measured (open circles) and calculated (solid curves) voltage V L ( t ) across the load resistance R L for four different waveforms (square (a, b), sawtooth (c), triangular (d), and sine wave (e, f)) at various frequencies. Concurrent high-speed video imaging allows the contact area A T ( t ) (see Fig. 6) to be measured from which C T ( t ) is calculated using equation (1). The solid curves, shown in Fig. 2 , represent the V L ( t ) values calculated using equation (2) with these calculated C T ( t ) values. All calculated numerical results for V L ( t ) agree well with the experimental measurements. 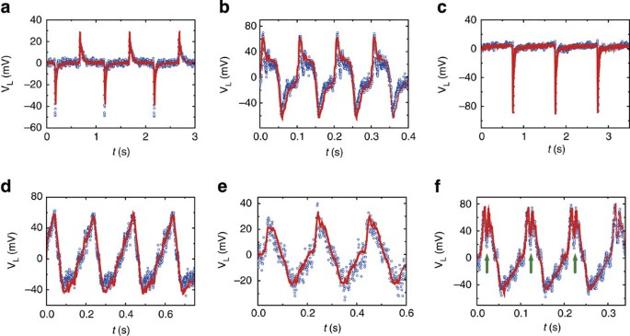Figure 2: Voltage dropVL(t) acrossRLas a function of timet. Experiment (open circles), numerical calculations using equation (2) (solid curves). Square wave inputs at (a)f=1 Hz and (b)f=10 Hz where the contact areaAT(t) increases sharply, stops and maintains its value for a half period, and then changes direction. (c) Sawtooth input atf=1 Hz whereAT(t) slowly increases linearly with time and then decreases sharply. (d) Triangular input atf=5 Hz. Sine wave inputs at (e)f=5 Hz and (f)f=10 Hz. For all graphs the droplet volumeV=40 μl and oscillation amplitudeL=0.5 mm. For (a–e)RL=10 MΩ and (f)RL=1 MΩ. Dips in (f) arise from an imperfect sinusoidal pattern inAT(t) (see arrows in Fig. 6f). Figure 2a show data for 1 and 10 Hz square wave input signals, respectively. At a low frequency ( Fig. 2a ), the voltage difference ΔV ( t ) becomes fully relaxed within a half period. However, at a high frequency ( Fig. 2b ), Δ V ( t ) has insufficient time to fully relax within a half period. Figure 2a , therefore, indicate that there is a close interrelationship between the vibration frequency and the relaxation time. Figure 2c exhibits data for a 1 Hz sawtooth input waveform. During the slow increase of A T ( t ), the relaxation occurs almost instantaneously at every moment and the value of V L ( t ) remains near zero, except at the very moment of a sharp decrease in A T ( t ). Figure 2d exhibits data for a 5 Hz triangular wave input signal. For a triangular input wave at a low frequency (for example, f =1 Hz), V L ( t )≈0. As f increases, V L ( t ) also increases. Figure 2e show data for 5 and 10 Hz sine wave input signals, respectively, (see Supplementary Movie S1). In Fig. 2a–f , all of the control parameters in the calculation of V L ( t ) are identical except for the oscillation frequency f and input signal pattern. Consequently, the same parameter values are used in the numerical calculations except for the value of the capacitance C T ( t ), which is calculated from the measured contact area A T ( t ). Figure 2: Voltage drop V L ( t ) across R L as a function of time t . Experiment (open circles), numerical calculations using equation (2) (solid curves). Square wave inputs at ( a ) f =1 Hz and ( b ) f =10 Hz where the contact area A T ( t ) increases sharply, stops and maintains its value for a half period, and then changes direction. ( c ) Sawtooth input at f =1 Hz where A T ( t ) slowly increases linearly with time and then decreases sharply. ( d ) Triangular input at f =5 Hz. Sine wave inputs at ( e ) f =5 Hz and ( f ) f =10 Hz. For all graphs the droplet volume V =40 μl and oscillation amplitude L =0.5 mm. For ( a – e ) R L =10 MΩ and ( f ) R L =1 MΩ. Dips in ( f ) arise from an imperfect sinusoidal pattern in A T ( t ) (see arrows in Fig. 6f). Full size image Dimensionless relaxation time From the observation of Fig. 2 , we can therefore define a dimensionless relaxation time, N , using two characteristic times: the RC relaxation time, τ, and the half-vibration period, T/2 . Even though the change in ΔV ( t ) originates from the change in C T ( t ), the relaxation process is the main driving force generating ΔV ( t ). The relaxation is a charge exchange process between two capacitors until V B =V T . Therefore, the ratio between the relaxation time and half-vibration period is a key factor determining ΔV ( t ). If N<< 1, that is, τ << T/2 , every change in V T ( t ) has sufficient time to decay away during time period T / 2 . Thus, the values of V T ( t ) and V B ( t ) are similar for much of T/2 which leads to a small V rms value (the root mean suqare value of V L ( t )). However, if N >>1, that is, τ >> T / 2 , there is insufficient time for complete relaxation, which gives rise to a large V rms value. In this later regime, an increase in N does not lead to a change in the value of ΔV ( t ) and thus V rms possesses a finite value. Hence, V rms increases with N for N <1, starts to saturate near N ~1, and remains constant for N >>1 (see Supplementary Fig. S1 ). As the dimensionless relaxation time N increases with f and R L , (see equation (4)), it is possible to verify the dependence of V rms on f and R L . The open circles (solid curve) in Fig. 3a show the experimentally measured (numerically calculated) V rms values at various frequencies, f , for a sine wave input. 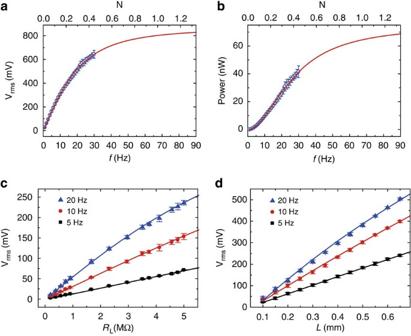Figure 3:Vrmsand power output under various conditions. (a)Vrmsand (b) power versus frequencyfandN, for a sinusoidal input, withL=0.6 mm andRL=10 MΩ. The vibration frequencyf~67 Hz corresponds toN~1. (c)VrmsversusRLfor three different input frequencies withL=0.6 mm. (d)Vrmsversus vibration amplitudeLfor three different input frequencies withRL=10 MΩ. Here, the droplet volume is 40 μl and the solid curves correspond to the numerical calculations. Data show mean±s.d. Figure 3b shows the electrical power generated for various frequencies. In this experiment, we only analysed data below 30 Hz because at high frequencies hydrodynamic effects deform the water bridge [18] , [19] . Figure 3c indicate that V rms increases approximately linearly with R L and L , respectively, for N <1 where, as the frequency f increases, V rms also increases. Figure 3: V rms and power output under various conditions. ( a ) V rms and ( b ) power versus frequency f and N , for a sinusoidal input, with L= 0.6 mm and R L =10 MΩ. The vibration frequency f ~67 Hz corresponds to N ~1. ( c ) V rms versus R L for three different input frequencies with L= 0.6 mm. ( d ) V rms versus vibration amplitude L for three different input frequencies with R L =10 MΩ. Here, the droplet volume is 40 μl and the solid curves correspond to the numerical calculations. Data show mean±s.d. Full size image Most small- or micro-scale electrical power generators for operating small electronic devices do not need large power output. Examples include chemical batteries [20] , [21] , [22] , solar cells [23] , piezoelectricity [24] , [25] , [26] , and thermoelectricity [27] . One important condition for the power generator is that at least a micro-Watt of power is required to operate such small devices [26] . In our system, however, Fig. 3b shows that the typical power of a single droplet is on the order of several tens of nW. Therefore, we need to find a way to increase the power output at least ten times. As the rate of change in A T ( t ) increases with the size of the water bridge, one can increase the power generated by increasing the volume of the water bridge. However, the size of the water bridge is limited by the capillary length of water, =2.7 mm. Here, g is the gravitational acceleration, ρ is the density of the fluid, and γ is the surface tension. A 40 μl water droplet corresponds to this capillary length. Therefore, if the volume of single droplet is larger than about 40 μl, the droplet no longer has a spherical cap shape and becomes pancake shape by the action of gravity [15] . As a result, the flattened droplet lowers the efficiency of the power generation. For a droplet size smaller than the capillary length scale, the power generation increases with the contact area. This difficulty can be overcome by forming numerous small and equally sized water bridges in parallel between the two plates. 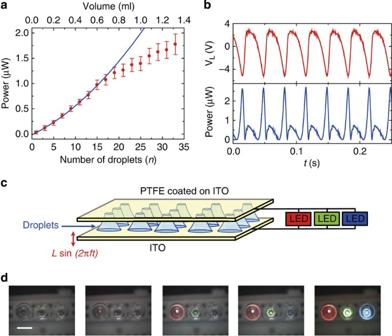Figure 4: Micro-watt power generation. (a) Power versus number of bridges for a sinusoidal input withf=30 Hz,L=0.6 mm andRL=10 MΩ (solid dots). Solid curve represents a parabolic fit. Volume of each single droplet is 40 μl. Data show mean±s.d. (b) Voltage dropVLand instantaneous power with time for the case of a 14 droplet system with the same conditions as (a). (c) Experimental setup for enhanced power generation. Three different LEDs are connected in parallel. (d) LEDs are lit up using 24 bridges for a sinusoidal input withf=30 Hz. Total volume of droplets is about 1 ml. Scale bar, 5 mm. The threshold voltage of the red, green, and blue LED is 1.8, 3 and 3.2 V, respectively. Figure 4a shows the electrical power generated depending on the number of bridges used (solid dots). As each bridge works as a current source, we expected that the power increases quadratically with the number of bridges (solid curve). However, this quadratic dependence of the power generation on the number of bridges starts to fail when the number of bridges is greater than 17. We believe that this deviation from a quadratic dependence originates from a desynchronization effect. The values of A T ( t ), from each bridge, do not synchronize with each other anymore, as the number of bridges increases, because all the liquid bridges cannot be made with exactly the same size and shape. This result demonstrates the potential of this method for practical applications. When the number of droplets is 14, the peak to peak voltage of V L is about 8 V and the instantaneous power is 0–3 μW ( Fig. 4b ). Figure 4c shows the experimental setup for micro-Watt power generation. Here, three different LEDs of red, green and blue colour, connected in parallel, are used as a load to confirm the practicality of our power generation system. In this experiment the vibration amplitude L is increased at a fixed vibration frequency of f =30 Hz. V L increases with vibration amplitude L . Figure 4d shows photo images of the three LEDs depending on V L . Red, green and blue LED lights are lit up one by one, in sequence, when V L is continuously increased. The threshold voltage for each LED differs. On the other hand, the LED lights go out in reverse order when V L is slowly decreased (see Supplementary Movie S2 ). Figure 4: Micro-watt power generation. ( a ) Power versus number of bridges for a sinusoidal input with f =30 Hz, L= 0.6 mm and R L =10 MΩ (solid dots). Solid curve represents a parabolic fit. Volume of each single droplet is 40 μl. Data show mean±s.d. ( b ) Voltage drop V L and instantaneous power with time for the case of a 14 droplet system with the same conditions as ( a ). ( c ) Experimental setup for enhanced power generation. Three different LEDs are connected in parallel. ( d ) LEDs are lit up using 24 bridges for a sinusoidal input with f =30 Hz. Total volume of droplets is about 1 ml. Scale bar, 5 mm. The threshold voltage of the red, green, and blue LED is 1.8, 3 and 3.2 V, respectively. Full size image The power output depends on the volume of water used. Water always evaporates in the air in natural condition. Therefore, the power output decreases with time due to the evaporation when the system is open to air. But when the system is properly airtight sealed, the power output does not change with time (see Supplementary Fig. S2 ). In this experiment, roughly 1 ml of water can generate about 1.5 μW of the power and the maximum power density (power generation per unit interfacial area) is 0.3 μW cm −2 . We believe that one can increase the maximum power density by changing the kind of liquid, controlling the concentration of salt inside the liquid, changing the material and the thickness of coating on the plates, and sealing the system completely in the near future. Humans can generate mechanical vibrations at low frequencies during daily life, for example, by walking, cycling and driving. In addition, vibration energy is provided by the most common machines like a fan, a CD player and a speaker. Therefore, it would be possible to apply this new scheme as an eco-friendly replacement for a battery or auxiliary power source in portable electronics, which require only small quantities of electrical power. Sample preparation As the voltage difference ΔV ( t ) increases with the thickness of the dielectric layer d (see equations (1) and (2)), the surface of the top plate was coated with a dielectric material using the spin-coating method. The top plate was made hydrophobic by spin coating a 1:10 Teflon (DuPont) and FC-40 (Fluorinert) mixture at 1,000 r.p.m. onto an ITO-coated surface. The FC-40 solvent was then removed by baking this coated glass plate in an oven at 180 °C for 1 day. The thickness of the Teflon-coated dielectric layer was determined to be ~300 nm using an Alpha-Step and SEM. The contact angles on the top and bottom plates were measured from the image of a droplet on the plate (40 μl). The contact angles for the ITO surface (bottom plate) and the Teflon-coated ITO (top plate) are 62.5° ( Fig. 5a ) and 107° ( Fig. 5b ), respectively, indicating that the surface of the top plate is more hydrophobic than the bottom one. 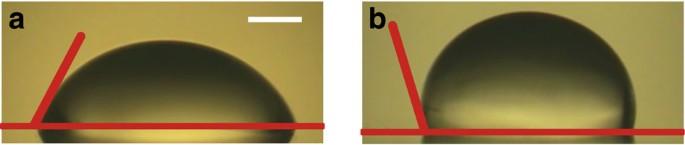Figure 5: Contact angle measurements. The image of a water droplet on the (a) ITO surface and (b) Teflon-coated ITO surface demonstrating their hydrophilic and hydrophobic properties, respectively. Scale bar, 1 mm. Figure 5: Contact angle measurements. The image of a water droplet on the ( a ) ITO surface and ( b ) Teflon-coated ITO surface demonstrating their hydrophilic and hydrophobic properties, respectively. Scale bar, 1 mm. Full size image Voltage measurements The signal input to the mechanical vibrator (V408, Ling Dynamic Systems, Inc), used to vibrate the bottom plate, was controlled using a power amplifier (EA200S, Elizer, Inc.) and function generator (33250A, Agilent, Inc.). The vibration amplitude, L , was measured using an accelerometer (353B16, PCB Piezotronics, Inc.) installed on the vibrating surface. The exact position of the top plate was precisely controlled by using a micromanipulator (5171, Eppendorf, Inc.). The voltages, V L ( t ) and V rms , on the load resistor, R L , were measured using an oscilloscope (TDS2014C, Tektronix, Inc.) and lock-in-amplifier (SR-830, Stanford Research Systems, Inc.), respectively. Numerical calculation The contact area on the top plate was imaged using a high-speed camera (SR-Ultra-C, Kodak, Inc.) at a frame rate of 250–500 per second where A T ( t ) was measured using a PC possessing image analysis software. The contact area, A T ( t ), is not exactly proportional to the input signal because of hydrodynamic flow in the water bridge, hydrophobic effects and imperfections in the surface condition of the top electrode. Consequently, when the bottom plate moves up (down), the rate of change of the top contact area is slower (faster) than expectations from the input oscillation signal. 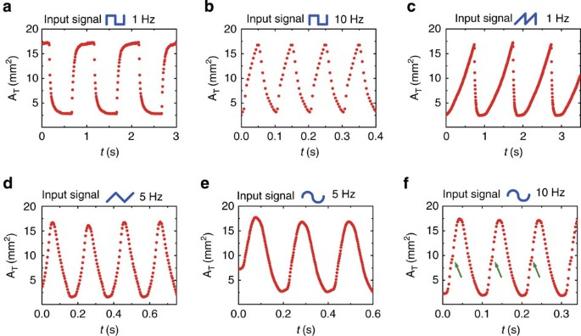Figure 6:AT(t) measurements using high-speed camera. There is a one-to-one correspondence betweenFig. 2andFig. 6. Figure 6a–f show the contact area A T ( t ) data used in the numerical calculation of the voltage drop V L ( t ) across R L as a function of time t in Fig. 2a–f . Figure 6: A T ( t ) measurements using high-speed camera. There is a one-to-one correspondence between Fig. 2 and Fig. 6 . Full size image The resistivity of fresh deionized water is about 18.2 Mohm cm −1 . In this case, the thickness of electrical double layer (the Debye length) λ D is 960 nm. However, deionized water in the lab, just before use, is not pure anymore because of exposure to the air and the electrodes. The measured resistivity of deionized water R f was about 2 Mohm cm −1 in this experiment. As we could not measure λ D , we used the value of λ D =300 nm from the previously published result by other researchers (see Table 3 in reference [16]) [16] . Therefore, using equation (1), the capacitances per unit area are C T / A T = ε 0 ε p / d =6.2 nF cm −2 and C B / A B = ε 0− ε d / λ D =230 nF/cm 2 . Here, ε p =2.1, ε d =78, d ~300 nm, and λ D ~300 nm. Therefore, contact areas < A T >~10 mm 2 and A B ~28 mm 2 correspond to < C T >~0.62 nF and C B ~64 nF, respectively. The numerical calculations of V L ( t ) were carried out using the Mathematica software, based on equations (1) and (2) using all the parameter values discussed above. How to cite this article: Moon, J.K. et al . Electrical power generation by mechanically modulating electrical double layers. Nat. Commun. 4:1487 doi: 10.1038/ncomms2485 (2013).